A mechanism-based inactivator of glycoside hydrolases involving formation of a transient non-classical carbocation The design of mechanism-based enzyme inactivators to generate chemical probes for biological research is an important challenge in carbohydrate chemistry. Here we describe the synthesis and biological evaluation of a novel carbocyclic mechanism-based inactivator of galactosidases (glycoside hydrolase families 27 and 36). Upon catalysis of this unnatural substrate, a transient non-classical carbocation forms within the enzyme active site. We show that the inactivation event, which proceeds via a bicyclobutonium ion intermediate, leads to a single alkylation event that occurs on the enzymatic nucleophile, an aspartic acid residue in this case. We also show that the catalytic proficiencies for enzymatic hydrolysis of substrates and inactivation by our bicyclo[4.1.0]heptyl analogue of galactose differ by only a factor of 20. This inactivator has the potential for further development as a useful biological research tool for both basic research and biotechnological applications. Glycoside hydrolases (GHs) are a broad group of enzymes that catalyse the hydrolysis of glycosidic bonds in a wide range of glycoconjugates. Growing awareness of the importance of GHs to fundamental biological processes, and of their utility in biotechnology, is stimulating interest in both identifying and modulating the activities of these enzymes. For application in biological samples in particular there has been increasing attention paid to developing techniques that capitalize on mechanism-based enzyme inactivators and their adaptation to generate activity-based probes [1] , [2] , [3] , [4] , [5] . The vast majority of GHs [6] catalyse a nucleophilic substitution at the anomeric carbon atom by stabilizing enzymatic transition states (TSs) that involve positive charge development on the anomeric carbon, which undergoes delocalization onto the endocyclic oxygen of the sugar ring [7] , [8] . GHs that catalyse reactions involving this sort of oxacarbenium ion-like TS use either a concerted (S N 2; shown for an α-galactosidase in Fig. 1a ) [9] , [10] or a stepwise (S N 1) [10] , [11] , [12] mechanism. Many GHs are tolerant to structural variation of the aglycone leaving group, and this enables their activities to be monitored using synthetic glycosides that incorporate chromogenic or fluorogenic leaving groups. However, with regard to the principal enzymatic recognition element—the pyranose glycone residue itself—functional group replacements such as changing hydroxyl groups to fluorine [13] or hydrogen [14] atoms generally result in significant loss of catalytic activity. The fluoroglycoside family of mechanism-based inactivators invariably require very good leaving groups (for example, dinitrophenolate or fluoride) to compensate for the substitution of a hydroxyl group by a fluorine atom [15] . Moreover, only a few GHs have been shown to hydrolyse substrates that contain a modified pyranose ring, in particular those in which the ring oxygen is replaced with a sulfur atom [16] , [17] , [18] . This sensitivity to structural variation within the pyranose ring arises from the critical need for charge delocalization within the TS by overlap of the endocyclic oxygen atom’s p-type lone pair with the developing positive charge at the nascent trigonal anomeric centre. 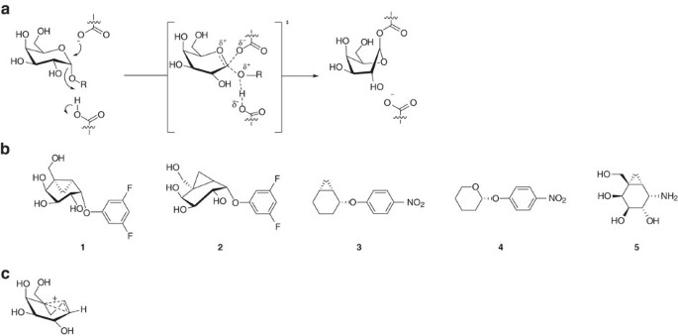Figure 1: Mechanism of glycosylation for retaining α-galactosidases from GH families 27 and 36, and structures of compounds. (a) First chemical step for a retaining α-galactosidase, which proceeds via an oxacarbenium ion-like TS to generate an enzyme bound intermediate. (b) Structures of the potential cyclopropyl-containing α-galactosidase inactivators (1and2), model compounds (3and4) and competitive α-galactosidase inhibitor (5) used in this study. (c) Postulated cationic intermediate formed from a cyclopropyl-containing ‘mechanism-based’ inactivator. Figure 1: Mechanism of glycosylation for retaining α-galactosidases from GH families 27 and 36, and structures of compounds. ( a ) First chemical step for a retaining α-galactosidase, which proceeds via an oxacarbenium ion-like TS to generate an enzyme bound intermediate. ( b ) Structures of the potential cyclopropyl-containing α-galactosidase inactivators ( 1 and 2 ), model compounds ( 3 and 4 ) and competitive α-galactosidase inhibitor ( 5 ) used in this study. ( c ) Postulated cationic intermediate formed from a cyclopropyl-containing ‘mechanism-based’ inactivator. Full size image The requirement for charge delocalization in GH catalysis led us to speculate that if we designed a substrate mimic that replaces the normal C–O acetal linkage with an unstrained exocyclic ether C–O bond, and that compound undergoes GH-catalysed hydrolysis, it would give a discrete carbocation within the enzyme active site. This cationic species would quickly react with nearby enzymic residues to yield an inactivated enzyme. Based on this idea and motivated by the high interest in ‘mechanism-based’ probes as tools in chemical biology [19] , [20] , [21] , [22] , we set out to develop a new class of inactivator that could show general applicability. We considered various carbocyclic-based carbohydrate mimics containing functionalities that are predisposed to form carbocationic intermediates during solvolysis reactions. After reviewing various options and taking into consideration the constrained active site structures of many GHs, we arrived at the key requirement that any structural changes made to the ring must be quite subtle. Keeping in mind that cyclopropylmethyl derivatives undergo S N 1 reactions at greatly accelerated rates [23] , [24] , [25] and that these reactions involve non-classical bicyclobutonium carbocation intermediates [26] , [27] , we therefore elected to evaluate the potential for constrained cyclopropyl σ-bonds to form cationic intermediates within the active site of GHs. Here we describe the synthesis of two bicyclo[4.1.0]heptyl analogues of galactose containing suitably strained σ-bonds that enable the enzyme-catalysed formation of cationic intermediates within the active sites of two retaining α-galactosidases from different GH families [6] . We define the extent of TS stabilization that these ‘mechanism-based’ inactivators receive from the enzyme and show that these compounds lead to covalent labelling of the enzyme within the enzyme active site at an essential catalytic residue. Synthesis of glycosidase inactivators We first synthesized bicyclo[4.1.0]heptyl-based D - galacto and L - altro analogues 1 and 2 ( Fig. 1b ), compounds that could generate the desired carbocationic intermediate ( Fig. 1c ), improving on a previous route [28] to obtain the known alcohol 6 from commercially available 2,3,4,6-tetra- O -benzyl- D -galactopyranose ( 7 ) in 15.0% overall yield ( Supplementary Methods and Supplementary Figs 1–5 ). We next achieved diastereoselective cyclopropanation of alkene 6 to obtain either 8 or 9 by including ~2 equivalents of trifluoroacetic acid in the reaction mixture [29] and by judicious choice of the reaction solvent. Nucleophilic aromatic substitution (S N Ar) of 1,3,5-trifluorobenzene [30] using each diastereomeric alcohol ( 8 and 9 ) enabled us to install a 3,5-difluorophenol or 3,5-difluorophenolate leaving group with the desired configuration at the pseudo-anomeric centre in yields of 68% and 75%, respectively ( Fig. 2 ). Following removal of the benzyl protecting groups by hydrogenolysis, we obtained the two bicyclo[4.1.0]heptyl carbohydrate analogues 1 and 2 . We assigned the relative stereochemistry of the two cyclopropyl compounds using 1 H NMR NOE difference experiments ( Supplementary Figs 6–9 ). 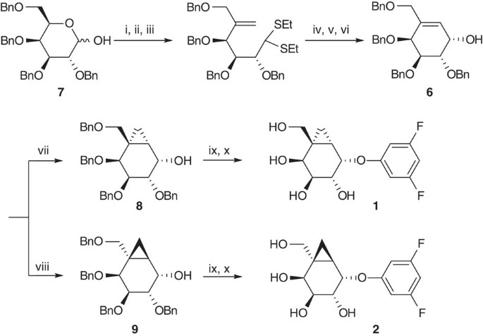Figure 2: Synthesis of carbocyclic analogues 1 and 2 of an aryl α-D-galactopyranoside. Reagents and conditions: (i) EtSH/HCl, 71%; (ii) oxidation, 87%; (iii) Ph3PCH2, 75%; (iv) HgCl2/H2O; (v) CH2CHMgBr in Et2O; (vi) Grubbs’ second-generation catalyst, 32% over three steps; (vii) ZnEt2, CH2I2, CF3CO2H in toluene, 79%; (viii) ZnEt2, CH2I2, CF3CO2H in dichloromethane, 78%; (ix) NaH, 1,3,5-trifluorobenzene in DMF; (x) H2/Pd-C (10%, w/w) in MeOH, over two steps 62% for1and 55% for2. Figure 2: Synthesis of carbocyclic analogues 1 and 2 of an aryl α- D -galactopyranoside. Reagents and conditions: (i) EtSH/HCl, 71%; (ii) oxidation, 87%; (iii) Ph 3 PCH 2 , 75%; (iv) HgCl 2 /H 2 O; (v) CH 2 CHMgBr in Et 2 O; (vi) Grubbs’ second-generation catalyst, 32% over three steps; (vii) ZnEt 2 , CH 2 I 2 , CF 3 CO 2 H in toluene, 79%; (viii) ZnEt 2 , CH 2 I 2 , CF 3 CO 2 H in dichloromethane, 78%; (ix) NaH, 1,3,5-trifluorobenzene in DMF; (x) H 2 /Pd-C (10%, w/w) in MeOH, over two steps 62% for 1 and 55% for 2 . Full size image Biological activity of α-galactopyranoside analogues 1 and 2 With these target molecules in hand, we first assayed the action of coffee bean α-galactosidase (a member of GH family 27 (GH27); for a review of the CAZy classification system, see ref. 31 ) with bicyclo[4.1.0]heptyl carbohydrate analogue 1 . We observed a time-dependent exponential decrease in enzymatic activity ( Fig. 3a ). We also found that the rate of inactivation decreased in the presence of the competitive inhibitor 5 (ref. 28 ), indicating that inactivation is driven by action occurring at the enzymatic active site ( Fig. 3b ). Analysis of the inactivation rate constants as a function of inactivator concentration reveals a hyperbolic curve in which the inactivation rate constant reaches a maximal value of k inact =5.6 × 10 –4 s –1 ( t 1/2 =20.6 min; Fig. 3c ). The simplest kinetic scheme consistent with these data is reversible binding of the inactivator to the enzyme active site to give a Michaelis complex (E:I). Stability of this complex is governed by a dissociation constant ( K i ) and a chemical inactivation step with a rate constant k inact ( Fig. 3d ). We note that the nonlinear fits of enzyme activity versus time ( Fig. 3a ) produced better fits when the activity at infinite time was not constrained to be zero, and we thus conclude that active enzyme is slowly being regenerated, as we show below in detail for the GH36 family α-galactosidase from Thermotoga maritima ( Tm GalA). We therefore include within this general kinetic scheme a first-order rate constant ( k react ) for reactivation of the enzyme. Interestingly, the L - altro isomer 2 showed no inhibition or inactivation of either coffee bean or T. maritima α-galactosidases at concentrations of up to 10 mM (data not shown), indicating that this compound either does not bind or fails to react within the active sites of these enzymes. 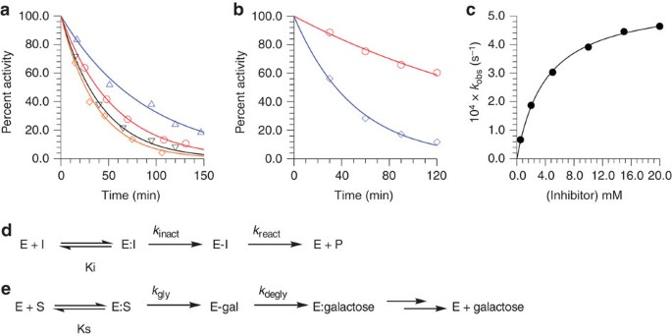Figure 3: Time-dependent inactivation of coffee bean α-galactosidase and kinetic schemes for GH27 and GH36 enzymes. (a) Concentrations of inactivator1are: (i) 20 mM (orange diamonds), (ii) 10 mM (black downward triangles), (iii) 5 mM (red circles) and (iv) 2 mM (blue upward triangles) in 50 mM phosphate buffer at a pH of 6.52 andT=37 °C. The coloured lines are the best nonlinear least squares fits to a standard first-order rate equation for the correspondingly coloured data points. (b) Decrease in coffee bean α-galactosidase activity during incubation with1(4 mM) in the presence (red circles) and absence (blue diamonds) of the competitive inhibitor5(1 μM) in 50 mM phosphate buffer at a pH of 6.52 andT=37 °C. (c) Michaelis–Menten kinetics for the inactivation of coffee bean α-galactosidase activity by1in 50 mM phosphate buffer at a pH of 6.52 andT=37 °C. The solid line shows the best fit of the data to a standard saturation kinetic expression. (d) Minimal kinetic scheme for inactivation of coffee bean α-galactosidase andTmGalA by1. (e) Kinetic scheme for both GH27 and GH36 enzyme families catalysed hydrolysis of α-galactopyranosides. Figure 3: Time-dependent inactivation of coffee bean α-galactosidase and kinetic schemes for GH27 and GH36 enzymes. ( a ) Concentrations of inactivator 1 are: (i) 20 mM (orange diamonds), (ii) 10 mM (black downward triangles), (iii) 5 mM (red circles) and (iv) 2 mM (blue upward triangles) in 50 mM phosphate buffer at a pH of 6.52 and T =37 °C. The coloured lines are the best nonlinear least squares fits to a standard first-order rate equation for the correspondingly coloured data points. ( b ) Decrease in coffee bean α-galactosidase activity during incubation with 1 (4 mM) in the presence (red circles) and absence (blue diamonds) of the competitive inhibitor 5 (1 μM) in 50 mM phosphate buffer at a pH of 6.52 and T =37 °C. ( c ) Michaelis–Menten kinetics for the inactivation of coffee bean α-galactosidase activity by 1 in 50 mM phosphate buffer at a pH of 6.52 and T =37 °C. The solid line shows the best fit of the data to a standard saturation kinetic expression. ( d ) Minimal kinetic scheme for inactivation of coffee bean α-galactosidase and Tm GalA by 1 . ( e ) Kinetic scheme for both GH27 and GH36 enzyme families catalysed hydrolysis of α-galactopyranosides. Full size image We observed that 1 inactivates Tm GalA at a much faster rate than it does the GH27 coffee bean enzyme, and, therefore, a more sensitive assay was needed for measuring enzyme activity ( Supplementary Table 1 ). Accordingly, we synthesized 6,8-difluoro-4-methylumbelliferyl α- D -galactopyranoside ( Supplementary Methods ), which gives large fluorescence changes upon hydrolysis. Using this substrate, we found that the half-life for reaction of the GH36 Tm GalA E:I complex is 49 s ( k inact =0.014 s −1 ), whereas that for the GH27 coffee bean enzyme is 20.6 min ( Supplementary Table 1 ). Given that the inactivation occurs relatively quickly and at the active site of the enzyme, we examined whether the inactivation process stems, as we expected, from covalent modification of Tm GalA. We therefore analysed both intact inactive enzyme and the active enzyme by electrospray ionization mass spectrometry (MS). A comparison of the reconstituted mass spectra of the native and the inactivated enzymes show a calculated mass difference between the major peaks in these two samples (172 Da), matching that expected for enzyme-catalysed cleavage of compound 1 and leading to single alkylation of the enzyme by the pseudo-carbohydrate portion of inactivator 1 ( Supplementary Fig. 10 ). Control experiments involving incubation of bovine serum albumin (BSA) with 1 showed no evidence for nonspecific alkylation of this protein (data not shown). Three criteria must be met for a compound to be a genuine ‘mechanism-based’ inactivator [32] . First, the reaction with the inactivator must occur within the confines of the enzymatic active site. Second, the enzyme must catalyse its own inactivation. Finally, the inactivator must be chemically unreactive before binding the target enzyme, whereupon it becomes activated and labels the enzyme [32] . This enhancement of reactivity within the enzyme active site can be considered as the ratio of the rate constants for 1 undergoing a spontaneous reaction to that for the enzyme-catalysed inactivation. To confirm that inactivator 1 meets the first criterion of a ‘mechanism-based’ inactivator, we identified the enzyme residue that is labelled during enzyme inactivation by 1 . That is, we incubated Tm GalA with excess inactivator and analysed, by electrospray ionization tandem MS (MS/MS), the tryptic peptides obtained by digestion of both the inactivated and the untreated enzyme ( Supplementary Methods ). Our analysis in positive ion mode revealed a tryptic peptide bearing a mass modification of 172.1 Da that corresponds to that of the pseudo-carbohydrate moiety of inactivator 1 minus a proton (172.1 Da). Fragmentation analysis revealed this peptide to be a 13-mer having the sequence ID*FLFAGAVPGER ( Fig. 4 ; asterisk indicates site of modification). The site of modification of T. maritima α-galactosidase by inactivator 1 is the nucleophilic aspartate residue (Asp327; Supplementary Fig. 11 ). We conclude that inactivation occurs through a chemical reaction at the enzyme active site since we find that: (i) Tm GalA is singly labelled and (ii) alkylation by the carbon skeleton portion of 1 occurs on an active site residue ( Fig. 4 ). These data unambiguously show that compound 1 meets the first criterion of a mechanism-based inactivator. 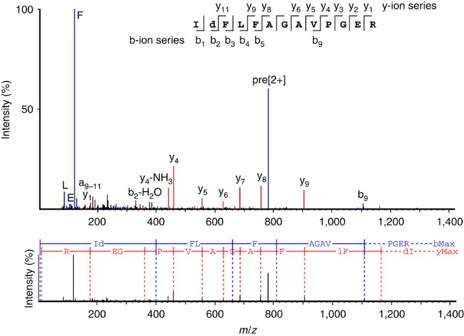Figure 4: Electrospray ionization tandem spectrometry (MS/MS) spectrum and analysis of the 13-mer peptide obtained by tryptic digestion of enzyme labelled with compound 1. The peptide sequence is noted at the top the MS/MS spectrum. The site of modification is denoted by the lowercase d in the peptide sequence shown at top. The doubly charged precursor ion is annotated as pre[2+]. The amino terminus-containing ions (b-ion series) are shown in blue and the carboxyl terminus-containing ions (y-ion series) are shown in red. These observed ions are noted beside the corresponding peaks in the MS/MS spectrum. Only major identified peaks are labelled for purposes of clarity. Figure 4: Electrospray ionization tandem spectrometry (MS/MS) spectrum and analysis of the 13-mer peptide obtained by tryptic digestion of enzyme labelled with compound 1. The peptide sequence is noted at the top the MS/MS spectrum. The site of modification is denoted by the lowercase d in the peptide sequence shown at top. The doubly charged precursor ion is annotated as pre[2+]. The amino terminus-containing ions (b-ion series) are shown in blue and the carboxyl terminus-containing ions (y-ion series) are shown in red. These observed ions are noted beside the corresponding peaks in the MS/MS spectrum. Only major identified peaks are labelled for purposes of clarity. Full size image Given that rapid labelling of Tm GalA occurs within the enzyme active site and this leads to a covalent adduct with the enzyme, we speculated that inactivation is catalysed by the enzyme itself. Both Tm GalA and the coffee bean enzyme are retaining galactosidases, hence they catalyse reactions using a two-step process involving the transient formation of a galactosyl enzyme intermediate ( Fig. 3e ) [33] . Two catalytic carboxyl groups play essential roles in catalysis, one as a general acid/base that assists the departure of the leaving group in the first step and attack of a water molecule in the second step, whereas the second carboxyl group acts as a nucleophile during glycosylation ( Fig. 1a ). The state of protonation of these residues is critical for effective catalysis. The catalytic activity of Tm GalA decreases at both low and high pHs, with apparent p K a values for ionization of the active site residues of 3.3 and 6.3, respectively [33] . To ascertain whether this probe meets criterion 2 and therefore depends on these two catalytic groups being in the appropriate protonation state for efficient inactivation by probe 1 , we monitored the rate of Tm GalA inactivation by 1 as a function of pH ( Supplementary Fig. 12a,b ). We found that the protonation state of the two active site aspartic acid residues affects, albeit less profoundly, the rate of galactosidase inactivation ( k inact / K i ) in a manner similar to that seen for the galactoside-catalysed hydrolysis of substrates ( k cat / K m ) [33] . Although these data are consistent with the idea that enzyme inactivation by 1 is aided by the catalytic machinery of Tm GalA, we were unable to fit our kinetic data to a ‘bell-shaped’ pH-rate profile because the small rate constant differences, which we measured between pH values of 3.2 and 8.9, resulted in ill-conditioned fits. Criterion 2 is therefore satisfied. In addition, we measured the dependence of the first-order rate constant for recovery of Tm GalA activity ( k react ) as a function of pH ( Supplementary Figs 12c and 13 ) and we calculated the values for the ratio of the two first-order rate constants ( k inact / k react ) as a function of pH ( Supplementary Table 2 ). The rate of reactivation for inactivated Tm GalA shows that one residue is needed in its protonated state to facilitate regeneration of active enzyme. Of note, the values for k inact / k react , which vary between 16 and 26, require that at steady-state conditions with saturating concentrations of inactivator over 94% of the enzyme must be present in the inactive alkylated form. Relative proficiencies for catalysis and inactivation Tm GalA has evolved to hydrolyse α-galactosides presumably through a defined reaction coordinate involving specific conformational changes in the pyranose ring [34] . The conformational requirements for formation of a cyclopropylmethyl carbenium ion (bicyclobutonium ion) are known. In particular, reactions that involve cyclopropyl σ-bond participation are controlled by stringent geometric requirements [26] , [35] , [36] , and efficient participation of a cyclopropyl C–C σ-bond requires the formation of a bisected geometry in the bicyclobutonium cation [35] , [37] . Indeed, in the case of the 2-cyclopropyl-2-propylium cation, this arrangement is 57 kJ mol −1 lower in energy than the perpendicular conformation [38] . Because the third criterion requires the enzyme to catalyse its own inactivation, we were interested in comparing the extent of TS stabilization provided by the enzyme for its inactivation by 1 with that for the catalysed hydrolysis of α- D -galactopyranosides. If the inactivation process efficiently exploits the catalytic machinery along a reaction pathway that mimics the enzyme’s action with normal galactoside substrates then the enzymatic proficiency for inactivation ( k inact / K i × 1/ k uncat ) will be large. The extremely slow rates of reaction for the spontaneous hydrolysis of carbohydrates ( t 1/2 for methyl α- D -glucopyranoside at 37 °C is estimated to be ~1.2 × 10 6 years) [39] make direct measurements impractical. We therefore used a surrogate system, making use of truncated model compounds 3 and 4 for estimating the relative rate constants for hydrolysis of galactopyranoside and inactivation by the bicyclo[4.1.0]heptyl inactivator 1 . Model compounds 3 and 4 do not contain electron-withdrawing hydroxyl groups, thus making their uncatalysed hydrolysis reactions occur on a measurable timescale [40] , [41] . Synthesis of 3 followed standard procedures ( Supplementary Methods ). As the reaction of 3 is still too slow to measure conveniently at 37 °C, we extrapolated the rate constant for this temperature from kinetic data acquired at higher temperatures ( Supplementary Table 3 ). The second-order rate constants ( k cat / K m and k inact / K i ) for the reactions of GH36 T. maritima α-galactosidase with 3,5-difluorophenyl α- D -galactopyranoside and the bicyclo[4.1.0]heptyl inactivator 1 , divided by the first-order rate constants for the spontaneous hydrolyses of model compounds 4 and 3 , respectively, gave enzymatic proficiencies for catalysis ( k cat / K m × 1/ k uncat ) and inactivation ( k inact / K i × 1/ k uncat ). Remarkably, these two enzymatic proficiencies differ by only a factor of 20, which indicates that the enzyme stabilizes the TS for substrate hydrolysis to a similar extent as the TS leading to formation of the bicyclobutonium ion (from reaction with 1 ), which then rapidly inactivates the enzyme (details provided in the Supplementary Table 4 ). Therefore, with regard to criterion 3, it is clear from the relative enzymatic proficiencies ( Supplementary Table 4 ) that Tm GalA promotes inactivation by bicyclic inactivator 1 by significantly lowering the TS-free energy for cleavage of the pseudo-glycosidic bond in 1 , a reaction that does not proceed at a measureable rate in the absence of the enzyme. Accordingly, we conclude that bicyclo[4.1.0] compound 1 satisfies all three criteria for being a bona fide ‘mechanism-based’ glycosidase inactivator. Notably, we find that Tm GalA-catalysed inactivation by 1 , which involves delocalization of positive charge onto a carbon skeleton ( Fig. 5a ), results in a decrease in TS stabilization free energy difference of only <8 kJ mol −1 when compared with that of the TS for the natural hydrolysis reaction catalysed by Tm GalA ( Fig. 1a ). As noted by Sinnott, a glycopyranosylium ion with a lone pair of electrons delocalized onto the cationic centre can only have four low energy conformations: 3 H 4 and 4 H 3 half-chairs and 2,5 B and B 2,5 boats [42] . When the conformational restriction is between C5 and C6, which in this case is a fused cyclopropyl ring, the four accessible conformations are the 3 H 2 and 2 H 3 half-chairs and the 1,4 B and B 1,4 boats. However, given that Tm GalA-catalysed inactivation involves a significant TS stabilization, we conclude that the reaction of 1 with the enzyme occurs from either a 3 H 2 half-chair or a 1,4 B boat conformation, as these are the two arrangements that possess the necessary bisected geometry for bicyclobutonium cation formation ( Fig. 5b ). Given the similar values obtained for the catalytic and inhibitive proficiencies for Tm GalA-catalysed reactions, one of these two ring conformations ( 3 H 2 or 1,4 B ) is likely to resemble the pyranose ring conformation at the enzyme-catalysed glycosylation TS [7] , [8] , although definitive support of this view awaits structural insights from complexes of these inactivators bound to enzymes. 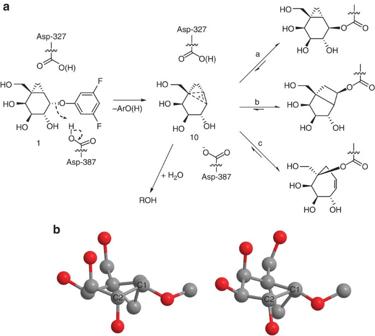Figure 5: Mechanism of enzyme labelling by the 'mechanism-based' inactivator 1 and conformational implications. (a), Postulated mechanism for inhibition of theT. maritimaα-galactosidase by the mechanism-based inactivator1. The dashed arrows to Asp-387 illustrate the possible role of this residue at the TS for carbocation formation. Asp327 is depicted in both protonation states, as the ionization state of this residue has only a small effect on the kinetics of inactivation. Bicyclic cation10could react, reversibly, to give cyclopropylmethyl (arrow a), cyclobutyl (arrow b) or homoallylic (arrow c) labelled Asp327 or it can react with water to give hydrolysed inactivator (ROH). (b) The two ring conformations for the bicyclo[4.1.0]heptyl inactivator1in which the C1–C2bond bisects the cyclopropyl ring (left:3H2half-chair; right:1,4B boat). Figure 5: Mechanism of enzyme labelling by the 'mechanism-based' inactivator 1 and conformational implications. ( a ), Postulated mechanism for inhibition of the T. maritima α-galactosidase by the mechanism-based inactivator 1 . The dashed arrows to Asp-387 illustrate the possible role of this residue at the TS for carbocation formation. Asp327 is depicted in both protonation states, as the ionization state of this residue has only a small effect on the kinetics of inactivation. Bicyclic cation 10 could react, reversibly, to give cyclopropylmethyl (arrow a), cyclobutyl (arrow b) or homoallylic (arrow c) labelled Asp327 or it can react with water to give hydrolysed inactivator (ROH). ( b ) The two ring conformations for the bicyclo[4.1.0]heptyl inactivator 1 in which the C 1 –C 2 bond bisects the cyclopropyl ring (left: 3 H 2 half-chair; right: 1,4 B boat). Full size image In particular, we propose that the intermediate generated by C–O bond cleavage of inactivator 1 is carbenium ion 10 ( Fig. 5a ). The mechanism presented in Fig. 5a shows three possible outcomes (reaction arrows a, b and c) [23] for trapping of the cationic intermediate 10 : formation of (a) a cyclopropylcarbinyl, (b) a cyclobutyl or (c) a homoallylic intermediate [23] , [36] . A detailed understanding of the pathway used by Tm GalA will be apparent once the structure of the covalent enzyme adduct is resolved. Reactivation of inactivated Tm GalA ( k react )—a process that is ~100-fold slower than its inactivation ( k inact )—likely involves the microscopic reverse of the inactivation reaction. This reversal would proceed via formation of carbenium ion 10 in the Tm GalA active site, and the cation then likely reacts with a water molecule to regenerate active enzyme. Although an electrophilic cation such as 10 could react with one of its hydroxyl groups, we view this possibility as unlikely given that within the active site all hydroxyl groups of bound substrates are involved in strong hydrogen-bonding interactions to enzymatic residues ( Supplementary Figs 14 and 15 ). In addition, we note that our cyclopropyl compound 1 inactivates the coffee bean α-galactosidase (GH27) while the corresponding 2-fluoro-α- D -galactopyranosyl fluoride shows no time-dependent inactivation [43] , and thus we suggest that cyclopropyl carbasugar inactivators maybe complementary to the 2-fluorosugar family of mechanism-based inactivators. In summary, based on the known chemistry of cyclopropylmethyl carbenium ions, which are generally (although not exclusively [44] ) viewed as non-classical bicyclobutonium ions [45] , we propose that enzyme inactivation by 1 occurs via the formation of a bicyclobutonium ion intermediate within the active site of the retaining galactosidase ( Fig. 5a ) from either a bound 3 H 2 half-chair or 1,4 B boat conformation ( Fig. 5b ). Subsequently, this intermediate is trapped by an Asp327, a reaction that follows the kinetically significant step, which is presumably cleavage of the C–O ether bond. To the best of our knowledge, this is the first example of a GH that reacts by producing a carbocationic intermediate that does not involve stabilization of positive charge development by a lone pair of electrons from an adjacent heteroatom. The resulting adduct is relatively stable and leads to inactivation of the enzyme. We speculate that other enzymes in which strained C–C σ-bonds are aligned to contribute to TS-positive charge delocalization will facilitate reactions within the enzyme active site to generate alkylated intermediates. We suggest that this structural motif for mechanism-based inactivation may have wide applicability because even when inactivation is slow, such as that seen for the reaction of the coffee bean enzyme by 1 , the inactivation rate constant ( k inact ) is expected to be increased, perhaps markedly, simply by changing the aglycone’s leaving group ability. Also, we suggest that the reactivation rate ( k react ) can be tuned to generate a more stable covalent adduct by substitution of a hydroxyl group. We propose that such modified compounds are likely to prove useful in studying GHs in various settings and could be valuable activity-based proteomics probes. Recombinant production of purified α-galactosidase We used a standard PCR technique to amplify the α -galactosidase galA gene from T. maritima MSB8 genomic DNA (American Tissue Culture Collection (ATCC) 43589D). The amplification media contained 5% dimethylsulphoxide, and the forward (5′-CGCGGCTAGCATGGAAATATTCGGAAAG-3′) and reverse (5′GCGCGAATTCTACCTGAGTTCCATCATTC-3′) primers encoded, respectively, NheI and EcoRI restriction sites (underlined), an alteration that changed the first codon of the gene from GTG to ATG. We purified the PCR fragment, and after digestion with NheI and EcoRI and insertion into the correspondingly digested pET28a vector (Novagen), the plasmid was introduced into Escherichia coli BL-21(DE3) by transformation. Plasmid DNA was isolated from a single bacterial colony, and it was verified using a restriction digest and DNA sequencing kit (Macrogen) with T7 promoter and terminator primers. The protocol used for expression and purification of Tm GalA was identical to that reported previously ( Supplementary Methods ) [46] . Enzyme kinetics We used 50 mM sodium phosphate buffer, pH 6.52, for coffee bean α-galactosidase inhibition assays. To determine the kinetic parameters K i and k inact for inhibition of both coffee bean and T. maritima α-galactosidases, we used a classical dilution assay method that involved incubating enzyme with various concentrations of inactivator ( 1 or 2 ) in the appropriate buffer and periodically measuring the activity of the enzyme by removing an aliquot (5 μl) of the inactivation stock solution and adding it to a solution of 4-nitrophenyl α- D -galactopyranoside (0.15 mM in 395 μl of 50 mM NaOAc buffer, pH=5.2; coffee bean enzyme) or 6,8-difluoro-4-methylumbelliferyl α- D -galactopyranoside (0.15 mM in 395 μl of 50 mM NaOAc buffer, pH=5.2; T. maritima enzyme). We determined pseudo first-order rate constants for inhibition ( k obs ) at each inactivator concentration by fitting the absorbance/fluorescence versus time data to a standard first-order rate equation (Prism 4.0). The first- and second-order rate constants ( k inact and k inact / K i , respectively) for the inactivation process were determined by fitting the k obs versus inactivator concentration data to a standard Michaelis–Menten expression. Reactivation kinetics In a typical enzyme reactivation assay, we added Tm GalA (40 μl, 1.2 mg ml −1 ) in 20 mM Tris-HCl buffer (pH 7.1) containing BSA (1% w/v) to a solution made by mixing aqueous Tris-HCl buffer (20 μl, 20 mM, pH 7.1) and a methanol solution of inactivator 1 (20 μl, 10.0 mM). After incubating the sample for 1 h at 37 °C, excess inactivator was removed and the inactivation buffer was exchanged by filtering the solutions using a 5-K molecular weight cutoff centrifugal filter and washing three times with reactivation buffer (3 × 300 μl) at 4 °C to give a final sample volume of 50 μl. Each of these samples was added to the appropriate buffer ( Supplementary Methods , pH-rate profile for inactivation section for a listing of buffers; final volume 300 μl) and incubated at 37 °C. We followed the α-galactosidase activity of each sample by periodically adding 5 μl aliquots of the reaction mixture to a cuvette containing a 37 °C solution of 6,8-difluoro-4-methylumbelliferyl α- D -galactopyranoside (3 μM) in NaOAc-HOAc-BSA buffer (50 mM, pH 5.2; 1% BSA) and monitoring the change in fluorescence (excitation 345 nM and emission 450 nm) using a Cary Eclipse Fluorescence Spectrometer. The measured initial rates were fit to a standard first-order rate equation to give estimates of the rate constant of reactivation ( k react ). Inactivation and labelling of α-galactosidase Incubation of Tm GalA α-galactosidase (50 μl of 0.4 mg ml −1 in 50 mM sodium acetate buffer, pH=5.2) with galacto -isomer 1 (1 mM) overnight at 20 °C was performed in parallel along with a negative control (no inactivator). We tested the activity of the enzyme samples as detailed above (reactivation kinetics section). After confirming that the inactivated enzyme had negligible activity relative to the control, we washed both samples (3 × 500 μl) with ammonium bicarbonate buffer (10 mM, pH 6.5) and submitted the samples for MS analysis. Details of site mapping can be found in the Supplementary Methods section. How to cite this article: Chakladar, S. et al. A mechanism-based inactivator of glycoside hydrolases involving formation of a transient non-classical carbocation. Nat. Commun. 5:5590 doi: 10.1038/ncomms6590 (2014).